Predator richness increases the effect of prey diversity on prey yield Positive biodiversity-ecosystem functioning relationships are generally attributed to two mechanisms: complementarity and selection. These mechanisms have been primarily examined using plant communities, whereas bacterial communities remain largely unexplored. Moreover, it remains uncertain how predation by single or multiple predators affects these mechanisms. Here using 465 bacterial microcosms, we show that multiple predation by protists results in positive bacterial diversity effects on bacterial yields (colony-forming units) possibly due to an increased complementarity and evenness among bacterial species. By mathematically partitioning the biodiversity effects, we demonstrate that competitive interactions in diverse communities are reduced and the growth of subdominant species is enhanced. We envisage that, including diversity gradients at other trophic levels, in biodiversity-ecosystem functioning research is a key to understanding and managing ecosystem processes. Such level of manipulation can be achieved best in microbial model systems, which are powerful tools for fundamental hypothesis-driven experiments and the investigation of general ecological theories. Identifying which ecological attributes of species affect the aggregate performance of a diverse ecosystem is instrumental for understanding the importance of biodiversity for ecosystem functioning [1] , [2] . Biodiversity-ecosystem function (BEF) theory suggests that positive biodiversity effects may arise mainly through two mechanisms referred to as ‘complementarity’ and ‘selection [3] , [4] , [5] . Complementarity is caused by either resource partitioning, niche differentiation, predator avoidance in mixtures or positive interactions among species. The selection effect describes the increasing probability of including a species with strong monoculture performance in species-rich experiments. Loreau and Hector [6] used a modified Price equation from evolutionary genetics [7] to partition these two effects whose composite or additive response determines whether, for example, the observed yield of diverse mixtures departs from the expected average of the monocultures yield (that is, the net biodiversity effect (NBE)). Fox [8] further developed a modified tripartite partitioning, which includes the three following mechanisms: the trait-independent complementarity (TIC; equivalent to the complementarity effect sensu Loreau and Hector [6] ) allows species to perform better in mixtures than in monoculture without reducing the average yield of other organisms in the mixture; the trait-dependent complementarity (TDC) is observed when changes in species’ performance are correlated with their traits (that is, monoculture yield), but also not at the expense of other species; and the dominance effect (DE) reflects pure competitive replacement at the expense of other species. The sum of DE and TDC equals the selection effect sensu Loreau and Hector [6] . The impact of trophic interactions (such as predation) on biodiversity effects still remains an understudied topic. The relatively few theoretical and experimental studies across trophic levels have shown quite complex BEF relationships, which are not captured by single trophic level observations [9] , [10] , [11] , [12] , [13] , [14] , [15] , [16] . Only a few studies have manipulated bacterial richness to reveal bacterial BEF relationships, [17] , [18] , [19] , [20] , [21] , [22] , [23] . However, it is in particular unknown whether richness effects at the higher trophic level interact with richness effects at the lower trophic level and how trophic interactions modify the above-mentioned three additive components (TIC, TDC and DE) along richness gradients. Although the majority of biodiversity-function experiments have focused on primary producers [24] , [25] , [26] , biodiversity effects are much less understood in bacterial communities. As predators strongly influence bacterial productivity, abundance and diversity [27] , [28] , it is of particular importance to understand the potential ecological effects and consequences of changing interactions among microbial trophic levels in the context of BEF research. We hypothesize that exposing bacterial communities to different predation pressures will change the direction and strength of bacterial interspecific interactions and result in different effects on productivity along the richness gradient. We further expect that predator diversity will affect the partitioning of the NBE into the three distinct mechanisms described above (TIC, TDC and DE), thereby casting light on the role of complementarity for the relationship between species richness and bacterial yield. Here we established five bacterial monocultures and all possible combinations of two to five bacterial species ( n =31) in microcosms ( n =465) and exposed them to three levels of predator diversity by three different bacterivorous protists (a flagellate, a ciliate and an amoeba). The bacterial strains and the three protists are common free-living microorganisms in various natural aquatic and soil ecosystems. The three predator species represent distinct modes of movement and predation such as flagellum-mediated filter feeding (the flagellate), cilium-mediated filter feeding (the ciliate) and surface gliding and feeding (the amoeba). We found that the impact of bacterial richness on bacterial yields and NBE in predation-free microcosms was constrained by dominance and negative complementarity effects. Although top–down control of bacterial richness effects in microcosms exposed to single predators was mostly nonsignificant and depended on predator identity, predation by multiple predators caused significant positive bacterial richness effects on yields possibly by increasing complementarity and bacterial species evenness. We suggest that strong richness yields relationships may rather emerge in systems with higher ecological complexity expressed in terms of species richness and interactions at both horizontal and vertical levels. Bacterial yields and NBE The observed bacterial yield (that is, colony-forming units (c.f.u)) and the NBE tended to increase as a function of bacterial species richness in all experiments ( Fig. 1 ). However, statistically significant positive relationships were obtained only in the presence of multiple predators (observed yield, P =0.006; NBE P =0.03; Fig. 1 ). Separate analyses of the bacterial community responses to the individual predator species demonstrated varying effects along the species richness gradient ( Fig. 2 ). In contrast to grazing by the flagellate Poterioochromonas sp. or by the amoeba Acanthamoeba sp., only the presence of the ciliate Tetrahymena sp. resulted in significantly lowered bacterial yield ( P= 0.001) and a tendency to lower NBE with increasing bacterial richness ( Fig. 2 ). 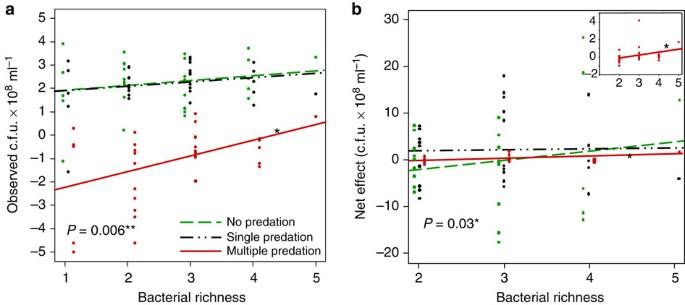Figure 1: Impact of different predation treatments on bacterial yields and NBE. Observed bacterial c.f.u (a) and NBE (b) as a function of bacterial species richness across all predation treatments and the predator-free control. Each point in the figure corresponds to the average of three replicates of each bacterial species combination. The points referring to treatments at equal richness are slightly offset horizontally for clarity. Results of the three single predator treatments are averaged. Statistically significant slopes are marked with ‘*’ and significance levels are given. The observed yield values are log transformed. The inside panel in (b) visualizes the NBE in microcosms exposed to multiple predation by spreading theyaxis. Figure 1: Impact of different predation treatments on bacterial yields and NBE. Observed bacterial c.f.u ( a ) and NBE ( b ) as a function of bacterial species richness across all predation treatments and the predator-free control. Each point in the figure corresponds to the average of three replicates of each bacterial species combination. The points referring to treatments at equal richness are slightly offset horizontally for clarity. Results of the three single predator treatments are averaged. Statistically significant slopes are marked with ‘*’ and significance levels are given. The observed yield values are log transformed. The inside panel in ( b ) visualizes the NBE in microcosms exposed to multiple predation by spreading the y axis. 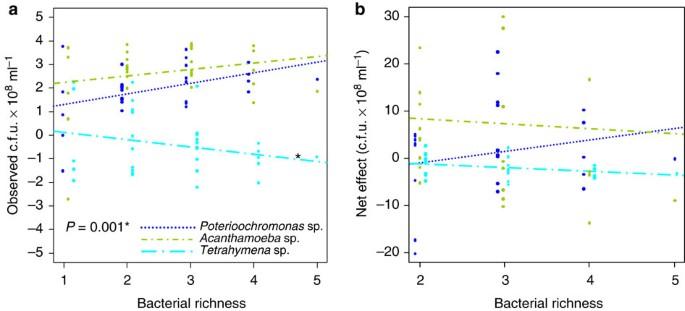Figure 2: Impact of predation by distinct single predators on bacterial yields and NBE. Observed bacterial c.f.u (a) and NBE (b) as a function of bacterial species richness in the single predator treatments. Each point in the figure corresponds to the average of three replicates of each bacterial species combination, and the points referring to each treatment are slightly offset horizontally for clarity. The observed yield values are log transformed. Statistical significant slopes are marked with ‘*’ and significant levels given. Full size image Figure 2: Impact of predation by distinct single predators on bacterial yields and NBE. Observed bacterial c.f.u ( a ) and NBE ( b ) as a function of bacterial species richness in the single predator treatments. Each point in the figure corresponds to the average of three replicates of each bacterial species combination, and the points referring to each treatment are slightly offset horizontally for clarity. The observed yield values are log transformed. Statistical significant slopes are marked with ‘*’ and significant levels given. Full size image Complementarity versus selection effects We further mathematically partitioned the NBE into its three mechanisms, namely TIC, TDC and DE [8] . Overall, statistically significant relationships between the three partitioned components and increasing bacterial richness were only observed in the multiple predation experiment: Complementarity (that is, TIC) strongly increased ( P =0.02), whereas the selection effect (that is, TDC and DE) decreased ( P =0.03 and P= 0.003) with increasing species richness ( Fig. 3a ). As for the observed yields and the NBE, responses of TIC, TDC and DE to individual single predators along the richness gradient differed and were nonsignificant ( Fig. 3b ). Analysis of the community level response across all levels of bacterial richness indicated an increase of complementarity under predation pressure ( Fig. 4 ). The TIC shifted from negative to positive in microcosms exposed to predation irrespective of predator identity and richness, whereas the effect size of competitive interactions (that is, DE) in microcosms comprising multiple predation was nearly zero. In the experiment without predation, DE was significantly higher from TIC and TDC. In microcosms exposed either to flagellate or amoeba predation no significant statistical difference was observed between TIC, TDC and DE. However, the presence of Tetrahymena sp. or multiple predators resulted in significantly higher TIC among bacterial species as compared with the selection effects (TDC and DE; Fig. 4 . ). As a consequence, the slope of evenness was highest in the multiple predation experiments ( Supplementary Fig. S1 ), implying that evenness increased with bacterial richness ( Fig. 5 ). The deviation between the relative c.f.u observed and the relative c.f.u expected for each individual bacterial species in species mixtures further showed that predation on diverse bacterial communities in fact caused a relatively better growth of less productive monocultures ( Supplementary Fig. S2 ). 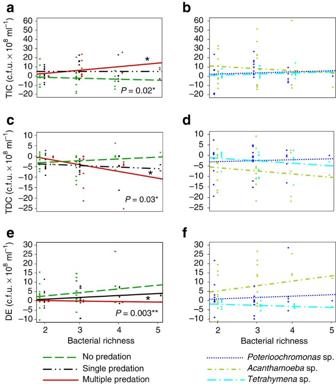Figure 3: Relationship between bacterial richness and the different components of NBE. (a,c,e) Responses of the three different components (TIC, TDC and DE) of the NBE as a function of bacterial species richness in all predation treatments and the predator-free control. Results of the three single predator treatments are averaged. (b,d,f) Responses of the three different components (TIC, TDC and DE) of the NBE as a function of bacterial species richness in all single predator treatments. The points referring to treatments at equal richness are slightly offset horizontally for clarity. Statistically significant slopes are marked with ‘*’ and significance levels are given. Figure 3: Relationship between bacterial richness and the different components of NBE. ( a , c , e ) Responses of the three different components (TIC, TDC and DE) of the NBE as a function of bacterial species richness in all predation treatments and the predator-free control. Results of the three single predator treatments are averaged. ( b , d , f ) Responses of the three different components (TIC, TDC and DE) of the NBE as a function of bacterial species richness in all single predator treatments. The points referring to treatments at equal richness are slightly offset horizontally for clarity. Statistically significant slopes are marked with ‘*’ and significance levels are given. 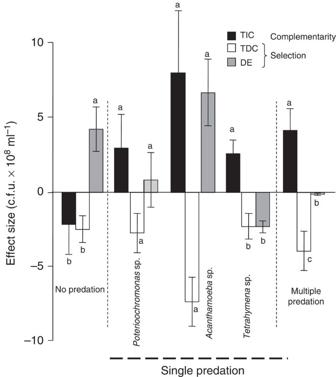Figure 4: Average effect size of NBE components across different predation treatments. Effect size of different biodiversity effects on yield in response to the different predator treatments across all diversity levels. Calculations are based on the tripartition approach9for each triplicate species combination in each individual treatment. Effects sizes represent average values for TIC, TDC and DE observed in each experiment and the bar represents standard error. The TDC and DE combined equal the selection effect, whereas TIC equals the complementarity effect of Loreau and Hector6. Letters on bars indicate statistical differences. Full size image Figure 4: Average effect size of NBE components across different predation treatments. Effect size of different biodiversity effects on yield in response to the different predator treatments across all diversity levels. Calculations are based on the tripartition approach [9] for each triplicate species combination in each individual treatment. Effects sizes represent average values for TIC, TDC and DE observed in each experiment and the bar represents standard error. The TDC and DE combined equal the selection effect, whereas TIC equals the complementarity effect of Loreau and Hector [6] . Letters on bars indicate statistical differences. 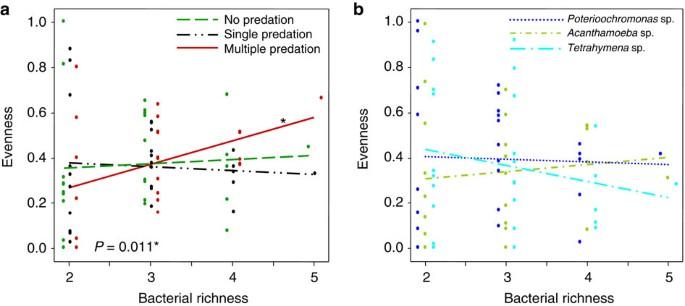Figure 5: Impact of predation on bacterial community evenness. (a) Bacterial community evenness as a function of bacterial species richness in all predation treatments and the predator-free control. Results of the three single predator treatments are averaged. (b) Bacterial community evenness as a function of bacterial species richness in all single predator treatments. Each point in the figure corresponds to the average of three replicates of each bacterial species combination. The points referring to treatments at equal richness are slightly offset horizontally for clarity. Statistically significant slopes are marked with ‘*’ and significance levels are given. Full size image Figure 5: Impact of predation on bacterial community evenness. ( a ) Bacterial community evenness as a function of bacterial species richness in all predation treatments and the predator-free control. Results of the three single predator treatments are averaged. ( b ) Bacterial community evenness as a function of bacterial species richness in all single predator treatments. Each point in the figure corresponds to the average of three replicates of each bacterial species combination. The points referring to treatments at equal richness are slightly offset horizontally for clarity. Statistically significant slopes are marked with ‘*’ and significance levels are given. Full size image In our microbial system, biodiversity effects tended to increase as a function of bacterial species richness in all experiments except in the microcosms with the predator Tetrahymena sp. The strongest and statistically significant results were observed for microbial communities exposed to multiple predators. Further, multiple predation resulted in the lowest bacterial yields of all treatments indicating a more substantial exploitation of prey resources ( Fig. 1 ). The top–down control of diversity effects not only depended on predator richness [13] , [29] , [30] but also on their identity ( Fig. 2 ), likely reflecting their different feeding modes, prey preferences and efficiencies [27] , [31] , [32] . Consequently, different predators should not be treated as one functionally substitutable trophic level. Among the three predators we used, the ciliate Tetrahymena sp. caused the most substantial reduction in bacterial yield and NBE along the bacterial species richness. The less pronounced negative effect of Tetrahymena sp. in the multiple predation treatment might be a consequence of its lower initial density relative to the single predator experiments. These results do not suggest a general relationship between bacterial (prey) diversity and predator effects and illustrate the difficulty to predict richness yield trajectories as a response of ecosystems to changes in trophic interactions and species richness. In a similar experimental manipulation of microcosm with four bacterial species and the ciliate predator Tetrahymena pyriformis , Jiang [20] also found a positive effect of diversity on bacterial community biovolume, but addition of the ciliate predator had no effect on diversity-functioning relationships in that study. Several other studies, however, reported that trophic interactions can alter these relationships: For instance, Duffy et al. [29] showed that grazer richness affected several ecosystem properties only in the presence of a higher-level consumer. Gamfeldt et al. [13] observed the strongest effects of prey diversity mainly at the higher consumer diversity. Moreover, positive biodiversity effects have been demonstrated to be disproportionately amplified when biotic disturbance by multiple predators is most intense [33] . Our multiple predation experiment also partly confirms theoretical work by Thébault and Loreau [11] , [12] , which predicts top–down control of an adjacent lower trophic level to cause a linear increase of total biomass with species richness. In the absence of predators, total prey yield may saturate at higher species richness levels as has also been predicted by previous studies [3] , [34] . By mathematically separating the NBE into its three mechanistic components, we found statistically significant relationships of these three mechanisms with increasing bacterial richness only in the multiple predation experiment. This indicates that strong richness yield relationships may rather emerge in complex ecological settings, but not in simplified ones. Overall, predation increased complementarity and decreased the selection effects in bacterial systems. The magnitude of these mechanisms along a bacterial richness gradient generally depended on predator identity ( Figs 3 and 4 ). The TIC shifted under predation from negative to positive, irrespective of predator identity and richness. A positive TIC indicates ‘mutual’ complementarity due to a better performance of all species when grown in mixtures [8] . This shift was accompanied by changes in DE, which became generally smaller in magnitude than TIC or even negative, whereas TDC was always negative regardless of predator treatment ( Figs 3 and 4 ). Negative values of DE and TDC reflect better growth in mixtures of species with low-monoculture yields at the expense of other species or without affecting other species, respectively. Contrary to most published studies to date [35] , [36] TDC contributed substantially to the observed responses in our microcosms. Fox [8] suggested that TDC effects arise from ‘nested niches’, if for instance niche overlap coincides with competitive release of subdominant species at altered diversity. Recent work on a plant–animal model suggests that nestedness emerges within a community if species experience minimal competition [37] . Such conditions may have been present in the multiple predator treatment, where we observed a strong TDC (that is, potential presence of nested niches) and a nearly zero DE (that is, minimal competition; Fig. 4 ), though an experimental proof that nested niches existed in our microcosms would require manipulating the range of conditions for niche separation. In experiments without predation, a positive DE indicated competitive species interactions by the most productive strain in multispecies mixtures ( Janthinobacterium sp., strain B3: Supplementary Fig. S2 a–1 ). Interestingly, the positive DE went along with a negative TIC, a rarely described phenomenon in BEF studies [25] , [26] ( Figs 3 and 4 ). The general dominance of Janthinobacterium sp. could be due to its capability to produce antimicrobial metabolites [38] that could suppress or reduce growth of other species in the mixtures. However, we did not observe any inhibition zone created by the used bacterial species. Additionally, negative TIC values hint at physical or chemical interference among species [6] , which are also common modes of interactions of bacterial communities in nature [39] . Overall, productive monocultures performed poorly in mixtures when no predators or only single predators were present ( Supplementary Fig. S2 ), explaining the nonsignificant biodiversity effects in these experiments ( Figs 1 and 2 ). Counteracting effects of complementarity and dominance or selection across a diversity gradient ( Fig. 3 ) are a rather common observation in diversity experiments [1] , [25] , [26] . As several resources were available as part of the culture medium (glucose, starch and amino acids) and all bacteria were capable of growing in the experimental media, we can only speculate about the axis of complementarity. In analogy to apparent competition [40] , the observed positive species complementarity may thus be interpreted as ‘apparent facilitation’ [41] , that is, predators tend to have a higher impact on the dominating prey, thus alleviating predation on some other bacterial species and allowing species with low-monoculture yields to perform better in mixtures. Our results support earlier theoretical arguments [11] that prey complementarity may arise from ‘predator partitioning’ rather than resource partitioning, that is, predators may be seen as a negative resource, where prey avoids the three predators differently, and hence complementarily. In the presence of predators preferring a single prey species, each bacterial species is controlled by its own predator and is unaffected by the addition of other species, which may also lead to a linear increase in complementarity effect [11] , [12] and decrease in DE ( Fig. 3a ). This phenomenon was most pronounced in the multiple predation experiments, where the effect size of competitive interactions was nearly zero (DE in Fig. 4 ). Consequently, microcosms comprising multiple predators resulted in higher bacterial species evenness across bacterial richness ( Fig. 5 and Supplementary Fig. S1 ). Even distribution of species has been shown to result in increased plant productivity with increasing species number [42] and predation-enhanced community evenness [28] , [43] is also considered an important mechanism of species coexistence in nature [44] . Additionally, a recent study with bacterial microcosms has also shown that an even initial distribution of community members ensures higher functional stability under selective stress conditions [45] . However, the role of evenness for the expression of interspecific interactions still deserves further attention, as some evidence with plant assemblages shows that neither complementarity nor selection necessarily changes with species evenness [46] . We acknowledge that our microcosm experiment simulates a rather low-richness community, in comparison with other microbial BEF studies [17] , [45] , and lacks several parameters that are often prevailing in field experiments, such as invasion, adaptation of predators and prey to each other or structural heterogeneity. Although our experimental design with colour-coded bacteria allows a mathematical separation of assumed interspecific mechanisms, we did not attempt to provide a direct physiological evidence for resource complementarity and facilitation. Future studies should now focus on an experimental manipulation of these mechanisms. Still, our study clearly demonstrates the importance of the trophic context for the BEF debate and the utility of microbial model systems for testing ecological hypotheses [47] , [48] , which may help in managing ecosystem processes. Bacteria as prey Five bacterial strains forming distinctly coloured colonies on the solid media applied ( Agrobacterium sp. B1, white colony colour), ( Micrococcus sp. B2, yellow), ( Janthinobacterium sp. B3, black), ( Williamsia sp. B4, pink) and ( Rhodococcus sp. B5, golden) were used in this study ( Supplementary Fig. S3 ). All bacterial strains have been deposited at the public Culture Collection of the Helmholtz Centre for Environmental Research –UFZ ( http://www.ufz.de/index.php?en=13354 ) and are available on request. All strains were maintained on Brunner CR-2 medium. The medium is a modified form of R2A complex medium, commonly used for cultivation of environmental bacteria [49] . The medium contained (g l −1 ): Na 2 HPO 4 (2.44), KH 2 PO 4 (1.52), MgSO 4 × 7H 2 O (0.2), CaCl 2 × 2H 2 O (0.01), NaCl (1.0), proteose peptone (0.25), yeast extract (0.25), tryptone (0.25), casamino acids (0.25), starch (0.5), glucose (5.0), (NH 4 ) 2 SO 4 (0.5), supplemented with vitamin solution (5 ml l −1 ) and trace element solution SL 10 (1 ml l −1 ) [50] . All strains grew on the medium selected. We intentionally used species with different growth characteristics (from best (B1, B3), to intermediate (B2, B5) to poorest performer (B4)). This in fact reflects typical ecological communities in nature in which species do not grow equally. Precultures were incubated for 25 h in closed Erlenmeyer flasks on a closed rotating shaker at 25 °C to assure actively growing cells. Depending on the growth of precultures, separate dilutions for each bacterial species were prepared in fresh medium to attain the required cell numbers in the microcosms. The total volume of microcosms consisted of 1.2 ml of liquid with an initial total bacterial density of about 2.11 × 10 7 bacterial cells, which was equal in all monocultures and mixtures. For the mixtures with differing species richness, dilutions were prepared and mixed accordingly to obtain maximum species evenness (that is, equal relative species abundance). Negative blank controls without organisms were used to assess contamination. Predation by protists Three protist species, that is, Acanthamoeba sp. (amoeba), Tetrahymena sp. (ciliate) and Poterioochromonas sp. (flagellate) were used as bacterivorous predators. Both Tetrahymena sp. and Poterioochromonas sp. were maintained in NSY (3 g l −1 ) [51] at 25 °C in an incubator without shaking. Acanthamoeba sp. was maintained in proteose–peptone–yeast–glucose medium [52] at 25 °C in an incubator without shaking. All strains were cultivated axenically (that is, growth on dissolved nutrients only without bacteria as food source) to avoid transfer of bacteria to the experiments. Protist cultures were grown in the respective media, concentrated by centrifugation [52] , [53] and washed with Brunner CR-2 medium before using them for the experiments. The overall total initial densities of protists were kept equal (5 × 10 4 cells) in all predator treatments. Experimental design We used a substitutive experimental design to test the impact of trophic interactions on bacterial diversity effects [6] . Previous BEF studies (for example, refs 17 , 22 ) used far more species, which were combined randomly into different diversity levels. In contrast, our experiment represents all possible combinations of the five species. The random-mixture-design runs the risk of obscuring species identity effects and mistaking them as diversity effects [54] , [55] . Our experimental design allows a statistical analysis that is unaffected by such identity bias (this is a special case of the sampling effect through design). In our full-factorial combination of species, every diversity level is independent of species identity. In random-mixture-designs one needs to correct, statistically, for species identity, which is usually not done. All possible combinations of monocultures and balanced mixtures of two to five bacterial species were established in 24-well microtiter plates (1.2 ml volume per well) with the same total initial bacterial density. The total initial density of bacteria and protist predators in monocultures and polycultures was thus the same at all richness levels. The experimental set up comprised three predator treatments: In experiment I, the five levels of bacterial species richness (one to five species) were established in the microcosms and incubated without predators. In experiment II, all bacterial richness levels were incubated with each of the three protist predators separately and in experiment III, microcosms were exposed to multiple predation pressure including all three predators together. The experiment comprised 155 microcosms in triplicates (465 in total). All communities were grown on Brunner CR-2 at 25 °C for 48 h without shaking. The yield (that is, c.f.u) of each bacterial species in each well was determined at the end of the experiments by quantifying the differently coloured bacterial colonies after plating on Brunner CR-2 agar plates. All visible colonies were recorded after 4 days of incubation at 25 °C using different dilutions from 10 −4 to 10 −8 thus allowing to calculate the relative abundance of different bacterial species in different combinations. Despite the frequent use of plant biomass as an ecosystem function, microbial biomass per se is not an appropriate indicator for ecosystem functioning. Moreover, c.f.u is not an ideal measure for total biomass as different strains have different cell volumes and physiological characteristics. Instead, we used the number of c.f.u as a measure for yield for two reasons: First, all strains were capable of growing on Brunner CR-2 agar plates and thus quantifiable after growth on these plates. Second, mathematically partitioning bacterial diversity effects requires determining the relative abundances of each species in each mixture (see data analysis below). Though defined community level microbial functions (for example, refs 17 , 22 ) could serve as a suitable proxy for ‘ecosystem functioning’, they cannot be assigned to individual species in a mixture. Counting differently coloured colonies was thus a rapid, easy and cheap approach to obtain the required yield data of each strain. Data analysis For each experiment, we calculated the average bacterial c.f.u after 48 h from triplicates for each bacterial combination on all richness levels. Biodiversity effects were analysed in term of log-linear plots [8] , that is, responses of c.f.u to changes in bacterial species richness were plotted after linear regression of log-transformed c.f.u values. Analysis of variance (ANOVA) analysis was done to determine the impact of bacterial species richness on the observed bacterial c.f.u. We applied Fox’s [8] tripartite equations to mathematically partition the observed bacterial diversity effects (c.f.u production as a proxy for yield) into its three different component mechanisms [8] : TIC, TDC and DE. This model was applied to every combination (in triplicate) of every experiment. This approach is a further modification of the additive partitioning developed by Loreau and Hector [6] for partitioning the NBE of multispecies assemblages. The NBE is the difference between the observed total yield and the expected total yield of a mixture under the null hypothesis that the intra- and interspecific interactions are identical. The observed total yield (that is, in our study c.f.u) of a multispecies mixture is the sum of the observed yields of all species in that mixture, whereas the expected total yield is the sum of the expected yields of each species present in that mixture, which are determined as the product of a species’ expected relative yield (the proportion in which it was seeded RY E below) and its yield in monoculture. In mathematical forms, the tripartite partition can be described as given below: Δ Y =NBE. N =no. of species in mixture. =average mass of all species in monoculture. RY O =observed relative yield of all species in the mixture. It is calculated by dividing its mass in mixture by its mass in monoculture. RY E =expected relative yield of all species in the mixture. It is the proportion in which a species is seeded or planted in mixture. =average deviation between RY O and RY E in the mixture. RYT O =sum of RY O of all species in the mixture. In the equation, the first part of the equation on the right side is the TIC. Similarly, the first covariance term in the above equation is TDC, and the last covariance term is DE. For details about this model, readers are advised to read the relevant literature [6] , [8] . ANOVA analysis was done to determine the impact of bacterial species richness on TIC, TDC and DE. In addition, ANOVA test followed by Tukey’s test was performed to determine the significance of differences among TIC, TDC and DE in different experiments. Pielou’s evenness J was calculated (as J =Shannon’s diversity index H/Hmax) on the basis of the obtained bacterial c.f.u from all bacterial communities at the end of the experiments. The resulting slope of evenness across bacterial diversity was calculated in all predation and no predation experiments. The deviation between relative yield observed and relative yield expected for an individual bacterial species in the mixture was calculated using Fox [8] to determine the difference between the performances of individual bacterial species when present in monoculture or in the mixture, respectively. How to cite this article: Saleem, M. et al. Predator richness increases the effect of prey diversity on prey yield. Nat. Commun. 3:1305 doi: 10.1038/ncomms2287 (2012).